Anatomically modern Carboniferous harvestmen demonstrate early cladogenesis and stasis in Opiliones Harvestmen, the third most-diverse arachnid order, are an ancient group found on all continental landmasses, except Antarctica. However, a terrestrial mode of life and leathery, poorly mineralized exoskeleton makes preservation unlikely, and their fossil record is limited. The few Palaeozoic species discovered to date appear surprisingly modern, but are too poorly preserved to allow unequivocal taxonomic placement. Here, we use high-resolution X-ray micro-tomography to describe two new harvestmen from the Carboniferous ( ∼ 305 Myr) of France. The resulting computer models allow the first phylogenetic analysis of any Palaeozoic Opiliones, explicitly resolving both specimens as members of different extant lineages, and providing corroboration for molecular estimates of an early Palaeozoic radiation within the order. Furthermore, remarkable similarities between these fossils and extant harvestmen implies extensive morphological stasis in the order. Compared with other arachnids—and terrestrial arthropods generally—harvestmen are amongst the first groups to evolve fully modern body plans. Despite the diversity of living harvestmen (Opiliones) [1] , their fossil record is sparse, and few Palaeozoic species have been described [2] . Nevertheless they represent one of the oldest groups of land arthropods. Devonian ( ∼ 410 Myr) harvestman fossils from the Rhynie Chert, while incomplete, preserve a three-dimensional internal anatomy suggestive of an essentially modern body plan [3] , [4] . In contrast other Devonian arthropods generally belong to extinct lineages. Well-preserved harvestmen are not recorded again until Cretaceous ( ∼ 100 Myr) ambers [5] . Other Palaeozoic records, including a long-legged fossil from the Early Carboniferous ( ∼ 340 Myr) of Scotland [6] , appear superficially modern, but remain too poorly preserved to allow an unequivocal resolution of their affinities. Recent studies have demonstrated the efficacy of applying μCT to three-dimensionally preserved, siderite (FeCO 3 ) hosted Carboniferous arthropod fossils [7] , [8] , [9] . Thus such concretions, common in the Euamerican Coal Measures, are among the most promising taphonomic windows for the high-fidelity preservation of Opiliones. Here μCT is used to describe two new harvestman species ( Ameticos scolos gen. et sp. nov. and Macrogyion cronus gen. et sp. nov.) from the Montceau-Les-Mines Lagerstätte ( ∼ 305 Myr), France, facilitating their inclusion into a phylogenetic analysis of living taxa using cladistic and probabilistic methods, and permitting inferences about the organisms' palaeobiology and mode of life. Systematic palaeontology of Ameticos scolos Class Arachnida Order Opiliones Sundevall, 1833 Suborder Dyspnoi Hansen & Sørensen, 1904 Ameticos scolos gen. et sp. nov. Etymology . From Greek, ametikos, of harvest and skolos, thorn. Holotype . Specimen MNHN-SOT 076167 (Collection Sotty 2, deposited in the Muséum d'histoire naturelle d'Autun) belonging to the Muséum national d'Histoire naturelle, Paris. ( Fig. 1a–c , reconstruction shown in Fig. 2 ., animation in Supplementary Movie 1 ). Locality, horizon and age . Montceau-les-Mines Lagerstätte (Massif Central, France), Assise de Montceau, Late Stephanian. Diagnosis . Dyspnoid harvestman with an elliptical body, broad prosoma/opisthosoma marked by ridge, and opisthosoma bearing three pairs of prominent spines. Cuticle ornamented with deep rounded pits. 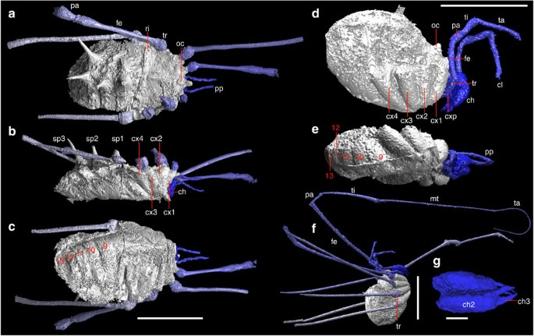Figure 1: Virtual fossils of Carboniferous Opiliones. Computer reconstructions of two new species of harvestman from the Stephanian Montceau-les-Mines Lagerstätte France. (a–c)A. scolosgen. et sp. nov. MNHM-SOT 076167. (a) Dorsal view. (b) Lateral view. (c) Ventral view. (d–g)M. cronusgen. et sp. nov. MNHM-SOT 079398. (d) Lateral view, walking legs removed and proximal pedipalps outlined. (e) Ventral view, walking legs removed. (f) Lateral view. (g) chelicerae, segments labelled. 9–13—segments 9–13; ch—chelicerae; ch 2–3—cheliceral segments 2–3; cx 1–4—coxae 1–4; fe—femur; mt—metatarsus; oc—ocularium; pa—patella; pp—pedipalps; ri—dorsal ridge; sp 1–3—dorsal spines 1–3; ta—tarsus; ti—tibia; tr—trochanter. Scale bar,a–c, 5 mm;d,e, 5 mm;f, 5 mm;g. 0.5 mm. Figure 1: Virtual fossils of Carboniferous Opiliones. Computer reconstructions of two new species of harvestman from the Stephanian Montceau-les-Mines Lagerstätte France. ( a – c ) A. scolos gen. et sp. nov. MNHM-SOT 076167. ( a ) Dorsal view. ( b ) Lateral view. ( c ) Ventral view. ( d – g ) M. cronus gen. et sp. nov. MNHM-SOT 079398. ( d ) Lateral view, walking legs removed and proximal pedipalps outlined. ( e ) Ventral view, walking legs removed. ( f ) Lateral view. ( g ) chelicerae, segments labelled. 9–13—segments 9–13; ch—chelicerae; ch 2–3—cheliceral segments 2–3; cx 1–4—coxae 1–4; fe—femur; mt—metatarsus; oc—ocularium; pa—patella; pp—pedipalps; ri—dorsal ridge; sp 1–3—dorsal spines 1–3; ta—tarsus; ti—tibia; tr—trochanter. Scale bar, a – c , 5 mm; d , e , 5 mm; f , 5 mm; g . 0.5 mm. 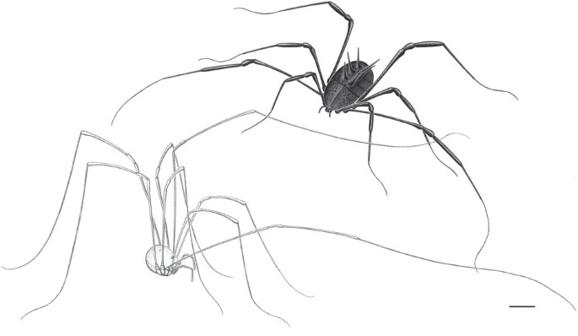Figure 2: Idealized reconstructions. The probable appearance in life ofA. scolosgen. et sp. nov. (above) andM. cronusgen. et sp. nov. (below). Scale bar, 5 mm. Full size image Figure 2: Idealized reconstructions. The probable appearance in life of A. scolos gen. et sp. nov. (above) and M. cronus gen. et sp. nov. (below). Scale bar, 5 mm. Full size image Description Large, elliptical body, 9.28 mm in length, prosoma/opisthosoma boundary with 0.49 mm thick, rectangular ridge ( Fig. 1a ). Dorsal surface well resolved, prosoma wide, flat and pitted towards the posterior. Subtle medial ridge runs from posterior to a small ocularium at anterior margin of carapace, drawn into a small projection. Left ventral surface heavily crushed, coxae of walking legs resolved on right ( Fig. 1b ), increasing in length from 1.87 mm (first) to 3.31 mm (fourth). Chelicerae small, three segmented, poorly resolved, total length 0.8 mm. Pedipalps also small, terminal claw not evident, either reduced or absent, podomeres tentatively identified as follows: femur 0.91 mm in length with distal apophysis, patella (0.46 mm), tibia (0.47 mm) and tarsus (0.47 mm). Most complete walking leg third left; trochanter 1.21 mm long, femur 6.07 mm, and bulbous, robust patella 1.38 mm. Femur proximally thin, but becomes bulbous towards the patella, longest in second limb despite premature truncation. Two walking legs (first and third right) truncate between trochanter and femur. Opisthosoma (5.68 mm long), bears three pairs of prominent spines 2.39 mm in length, resulting dorso-ventral maximum thickness 5.12 mm. Five tergites resolved (1: 1.21 mm long, 2: 1.15 mm, 3: 1.80 mm, 4: 0.89 mm, 5: 0.80 mm), first three bearing two spines per somite. Surface strongly ornamented with spherical pits, 0.23 mm in diameter. Five sternites visible ( Fig. 1c , numbered 9–13), first (9) longest, but anterior extent unclear. Next four well resolved, decreasing in size posteriorly. Systematic palaeontology of Macrogyion cronus Suborder Eupnoi Hansen & Sørensen, 1904 Macrogyion cronus gen. et sp. nov. Etymology . From Greek makros, long + gyion, limb and Cronus/Kronos, father of Zeus, Hades and Poseidon, and god of the harvest. Holotype . Specimen MNHN-SOT 079398 (Collection Sotty 2, deposited in the Muséum d'histoire naturelle d'Autun) belonging to the Muséum national d'Histoire naturelle, Paris. (MNHM 079398, Fig. 1d–g , reconstruction shown in Fig. 2 , animation in Supplementary Movie 2 ). Previously figured by Dunlop [10] . Locality, horizon and age . Montceau-les-Mines Lagerstätte (Massif Central, France), Assise de Montceau, Late Stephanian. Diagnosis . Eupnoid with mid-prosomal ocularium, palp tibia bearing distal apophysis and a bi-lobed ridge on dorsal opisthosoma. Description Oval body 6.53 mm in length, prosoma/opisthosoma boundary indistinct ( Fig. 1d ). Third left coxa and opisthosoma partially crushed, cuticle poorly resolved, likely thin and leathery in life. Maximum dorso-ventral thickness 5.88 mm. Robust three-segmented chelicerae well preserved, between pedipalps ( Fig. 1g ); first segment 0.93 mm in length, second 1.78 mm, and distal segment 0.62 mm forming the chela. Gracile pedipalps well preserved, held aloft and in front of the prosoma. Terminal apotelic claw. Podomeres (lengths) are tarsus (2.59 mm), tibia (1.09 mm) with distal apophysis, patella (0.83 mm), femur (1.73 mm), trochanter (1.02 mm), and coxa (0.52 mm). Walking legs elongate ( Fig. 1f ), first left preserved in its entirety—coxa, trochanter (0.95 mm in length) and femur (1.77 mm) orientated dorsally. Limb bends to a sub-horizontal patella (2.17 mm long), followed by ventrally orientated tibia (7.07 mm), and metatarsus (14.46 mm). Curved, highly annulated tarsus (10.65 mm in length), tarsomeres poorly resolved. Third left walking leg ventrally orientated from trochanter, preserving a small portion of a disarticulated coxa, trochanter (0.81 mm long), femur (14.57 mm), patella (2.34 mm), and tibia (6.93 mm). Truncated mid-metatarsus. All other limbs directed dorsally and truncated to top of femur, with exception of first right truncated post-patella. Prosoma slightly distorted, 3.22 mm wide, with mid-prosomal medial ocularium, triangular in section, eyes and ozopores not resolved. Coxae well preserved, increasing in size posteriorly from 2.00 mm (coxa 1) to 2.35 (coxa 4). Intercoxal region marked by medial groove but poorly resolved. Opisthosoma (4.86 mm) smooth, dorsal segments fused before three visible at posterior. Anterior dorsal opisthosoma bears a small bi-lobed ridge. Ventral opisthosoma with five clear sternites ( Fig. 1e , numbered 9–13), anteriormost significantly longer (0.96 mm) than those that follow (0.6–0.7 mm). Phylogenetic analyses Parsimony analysis of the unweighted morphological characters in TNT [11] using a driven search strategy with SPR, TBR and tree fusing and asking to retrieve minimum tree length 1,000 times yielded 217 trees of 225 steps. The strict consensus of these trees finds monophyly of Opiliones, Cyphophthalmi, Phalangida, Opilionidae, Hesperonemastoma + Sabaconidae, Laniatores as well as some structure within Cyphophthalmi and Laniatores. The fossil taxa are resolved as part of Phalangida, but their exact position is unresolved. Exclusion experiments with the two new fossils are interesting. When no fossils are analysed (or only with Halitherses included), all four suborders are recovered with a topology compatible with those from the previous studies. The addition of M. cronus causes collapse of Eupnoi, whereas the addition of A. scolos causes collapse of Dyspnoi. In no case does M. cronus appear within Dyspnoi or Laniatores nor does A. scolos nest within Eupnoi or Laniatores. Symmetric resampling ( P =33) fails to find a supported position for the fossils (2% for the inclusion of M. cronus within Eupnoi; 15% for the placement of A. scolos in Dyspnoi; 42% for Phalangida including the fossils). It is clear that the amount of missing data in key characters for resolving internal Opiliones phylogeny has a negative effect in this data set. Analysis of the same data set under implied weights [12] using a k =3 yielded 50 trees with a best score of 13.01429, but this tree is identical to that of the unweighted analysis. This tree is stable to variations in concavity values ( k =1, 85 trees, 21.9833 steps; k =10, 96 trees, 5.57160 steps), but higher k values have an effect in resolving Dyspnoi, including M. cronus and Halitherses ( k =100, 26 trees, 0.68163 steps), however, symmetric resampling was low for the membership of M. cronus to Eupnoi and of A. scolos to Dyspnoi. The morphological data set was combined with the molecular data set of ref. 13 to test whether the monophyly of Eupnoi and Dyspnoi, strongly supported by the molecular data, had an effect on the stabilization of the fossil taxa. Analyses under equal weights (2,031 steps), 3211 (2,935 weighted steps), 3221 (3,946 weighted steps)) assign M. cronus to Eupnoi and A. scolos to Dyspnoi ( Fig. 3 ). The NEXUS file for this is provided as Supplementary Software 1 . 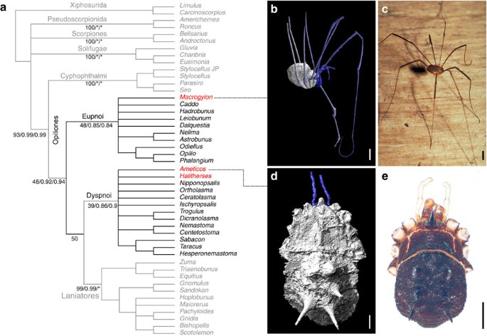Figure 3: Phylogenetic placement of fossils. (a) A cladogram of fossil and Recent harvestmen, derived from the dataset of refs5,13analysed in POY under direct optimization, showing the position ofAmeticos scolosgen. et sp. nov. andMacrogyion cronusgen. et sp. nov as members of the suborders Dyspnoi and Eupnoi, respectively. Numbers at nodes indicate jackknife frequencies/posterior probability of the implied alignment analysed in MrBayes/posterior probability of the MAFFT alignment analysed in MrBayes—further details of cladistics can be found in the Methods. Fossil-only taxa represented in red. Images on right showb,M. cronusandd,A. scoloswith comparable taxa of the modern Eupnoi and Dyspnoi;c,Nelima sempronii, Sclerosomatidae and e,Acuclavella cosmetoides, Ischyropsalididae. (c) courtesy of Christian Komposch, Ökoteam, Graz; (d) courtesy of Casey Richart, San Diego State University. Scale bar,b,c, 2 mm;d,e, 1 mm. Figure 3: Phylogenetic placement of fossils. ( a ) A cladogram of fossil and Recent harvestmen, derived from the dataset of refs 5 , 13 analysed in POY under direct optimization, showing the position of Ameticos scolos gen. et sp. nov. and Macrogyion cronus gen. et sp. nov as members of the suborders Dyspnoi and Eupnoi, respectively. Numbers at nodes indicate jackknife frequencies/posterior probability of the implied alignment analysed in MrBayes/posterior probability of the MAFFT alignment analysed in MrBayes—further details of cladistics can be found in the Methods. Fossil-only taxa represented in red. Images on right show b , M. cronus and d , A. scolos with comparable taxa of the modern Eupnoi and Dyspnoi; c , Nelima sempronii , Sclerosomatidae and e, Acuclavella cosmetoides , Ischyropsalididae. ( c ) courtesy of Christian Komposch, Ökoteam, Graz; ( d ) courtesy of Casey Richart, San Diego State University. Scale bar, b , c , 2 mm; d , e , 1 mm. Full size image Analysis of molecular data only in MrBayes yielded a topology compatible with the POY tree presented by ref. 1 , with Laniatores as sister group to all other Opiliones and Cyphophthalmi as sister group to Palpatores. This result is interesting, as both the data sets and analyses are very different between these two publications. Support for the suborder relationships are, however, low, although Opiliones and each suborder receive a posterior probability of 1.00. The analyses of the combined data set of morphology and molecules in MrBayes supported the more traditional view, with monophyly of Opiliones, Phalangida, and Palpatores, suggesting that the addition of the morphology has a positive impact with respect to the molecular data alone. When the fossils were added to the analyses, the topology was identical, and in both alignments (implied alignment from POY and MAFFT) Macrogyion was placed with Eupnoi and Ameticos with Dyspnoi, however, PP values are below 0.95 (0.84 and 0.85 for Macrogyion within Eupnoi in the MAFFT and implied alignment analyses, respectively; 0.90 and 0.86 for the placement of Ameticos [and Halitherses ] in Dyspnoi—see Fig. 4 ). 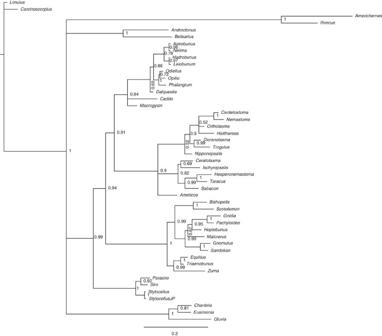Figure 4: Phylogram of fossil and Recent harvestmen. This is derived from the dataset of refs5,13analysed with MrBayes, and shows the position ofAmeticos scolosgen. et sp. nov. andMacrogyion cronusgen. et sp. nov as members of the suborders Dyspnoi and Eupnoi respectively. Numbers at nodes indicate posterior probabilities. Figure 4: Phylogram of fossil and Recent harvestmen. This is derived from the dataset of refs 5 , 13 analysed with MrBayes, and shows the position of Ameticos scolos gen. et sp. nov. and Macrogyion cronus gen. et sp. nov as members of the suborders Dyspnoi and Eupnoi respectively. Numbers at nodes indicate posterior probabilities. Full size image We also evaluated the residual trees evaluated by MrBayes, and in no case did Ameticos fall outside Dyspnoi. In the case of Macrogyion , there is only one conflicting topology, placing it with Dyspnoi instead of Eupnoi ( PP =0.084), a value that is significantly worse than the only other alternative, its placement with Eupnoi ( PP =0.84). All analyses therefore support the same placement of the fossils. In conclusion, most analyses assign M. cronus to Eupnoi and A. scolos to Dyspnoi, whereas no alternative position is significant for any method of alignment or data analysis. While confidence is low, the results suggest placement in the above suborders rather than in any of the others. The presence of an ocular tubercle and lack of ozophores clearly identifies the two fossils as members of Phalangida, but preservation does not allow for the identification of the eyes. Although M. cronus clearly belongs to the clade Phalangioidea in the suborder Eupnoi, the synapomorphy that delimits the clade, the accessory tracheal spiracles on the tibiae of the pedipalps and legs [14] , is not observable in the fossil specimen. Dyspnoi are characterized by the presence of diaphanous cheliceral teeth, the lack of a palpal tarsal claw, and for having a palpal tarsus shorter than the tibia. Preservation of the chelicerae does not allow for distinction of the teeth, and, although the lack of a palpal claw is inferred from the reconstruction, podomere delimitation is uncertain. Therefore, the lack of the claw is the only character that could identify Ameticos scolos as a member of Dyspnoi. Other characters such as the forwardly projecting ocularium or the dorsal spination resemble those of the genus Acuclavella , but this was not included in the matrix. Genitalic characters, which constitute the basis for most of the taxonomy within these clades, are not available for either fossil. The relatively complete and high-fidelity preservation of these new species has allowed the first cladistic analysis of any Palaeozoic harvestmen. Extant Opiliones can be divided into four major suborders, the Eupnoi, Dyspnoi, Laniatores and Cyphophthalmi. The phylogenetic trees derived from combined analysis of morphological and molecular data under parsimony direct optimization and Bayesian phylogenetics place Ameticos with Dyspnoi, and Macrogyion with Eupnoi ( Fig. 3 ). The presence of Eupnoi in the Devonian Rhynie fauna has previously been inferred on the basis of preserved genital morphology [4] , but the confirmation of a Carboniferous eupnoid, using a much broader set of characters, adds weight to suggestions that this is an ancient suborder. Ameticos is the earliest dyspnoid (but see phylogenetic analysis for details). Despite a residual level of uncertainty, this is the only dyspnoid from the era to be cladistically placed; contemporaneous taxa have only very tentatively been assigned to the clade [15] , [16] on the basis of gross morphology, and some may be misinterpreted eupnoids [2] (for example, the extinct family Nemastomoididae [17] ). The earliest hitherto described dyspnoid is Late Cretaceous in age [5] , thus Ameticos pushes the group's earliest appearance back significantly. These fossils hence corroborate recent molecular work [1] that postulates an Early Devonian origin for both the Dyspnoi and Eupnoi, and furthermore, offer new, robust calibration points for future studies of this nature. By the Late Carboniferous arachnids, such as spiders and scorpions, are largely known from their most basal lineages or from their stem forms [18] , only Palaeozoic mites [19] , [20] possess a similarly modern habitus. The presence here of two extant harvestman suborders provides compelling evidence for early Palaeozoic cladogenesis in the Opiliones. Despite their antiquity, both Montceau harvestmen are essentially modern in appearance, demonstrating that Opiliones' body plans were established by the Late Carboniferous and have remained largely unchanged in the 305 million years since. This old age and high degree of evolutionary stasis, coupled with a low vagility, further highlights the Opiliones' importance as a model for studying biogeographical patterns and evolutionary processes [21] . A. scolos bears a striking resemblance in all aspects of its morphology to certain living members of the Dyspnoi; most notably ischyropsalidids of the genus Acuclavella [22] ( Fig. 3 ). Furthermore we can infer behavioural similarities; using femoral length as a proxy for leg length, Ameticos would have had elongate second walking limbs, serving a tactile and sensorial function, as with Acuclavella (and a number of other modern harvestmen). Heavy surface ornamentation suggests a robust, well-sclerotized cuticle (exoskeleton), and implies a ground (rather than canopy) dwelling ecology. Acuclavella cosmetoides lives at the margins of small perennial water features in moist, woody debris (ref. 22 and C. Richart, personal communication); its spines may provide defence against amphibian predators. Ameticos could have inhabited similar regions in the moist, detritus-rich Carboniferous coal forests, and likely bore spines for the same reasons. A superficially similar habitus is also seen in Eupnoi of the genus Astrobunus , for example, A. laevipes. This species lives in the leaf litter of riparian and deciduous forests [23] , further supporting such speculation. M. cronus is similarly comparable to modern eupnoids in the families Phalangiidae and Sclerosomatidae, even down to fine details such as the limb podomere proportions, body shape/size, and the anterior appendages. The body of the fossil is partly crushed and less well preserved than the limbs, which implies soft and leathery cuticle comparable to modern eupnoids. The single complete leg possesses a highly annulated (subsegmented) tarsus, allowing a smooth curve at the limb's termination, another condition typical of extant eupnoids, and a possible adaptation towards life in vegetation that facilitates grip on plant stems through the formation of coils at the end of the legs [24] . Highly elongated limbs in many members of the Eupnoi are also indicative of life above ground level [24] ; we thus suggest a vegetation-dwelling or possibly arboreal ecology for Macrogyion . Materials Two fossils from Montceau Les Mines, MNHN-SOT 079398 and MNHN-SOT 076167 were selected. Both are hosted within small siderite nodules, MNHN-SOT 079398 is void, whereas MNHN-SOT 076167 appears to be infilled with kaolinite—only the posteriormost opisthosomal spines and a cross-section of the fossil are visible in the cracks splitting the nodule. X-ray micro-tomography Both specimens were scanned at the Natural History Museum, London on a Metris X-Tek HMX-ST, with a current/voltage of 190μA/180 kV, an unfiltered tungsten reflection target, and 3142 projections, giving a resolution of 26.5 μm. (MNHN-SOT 079398) and 14.2 μm (MNHN-SOT 076167). The resulting parallel slice images of the fossils allowed three-dimensional, virtual models of organisms to be created using the custom SPIERS software suite [25] . All pixels darker than a user-defined grey-level were assumed to belong to the fossil, through the creation of inverted linear threshold images. Manual cleaning was used to remove artefacts where pixels had been incorrectly identified as fossil or matrix, and then the images were masked. Regions of interest for individual anatomical features were defined through the use of a spline-based curve system, allowing them to be rendered as separate isosurfaces, and facilitating the removal of cracks from the model. The isosurface-based 3D models were inspected to allow iterative improvement of the regions of interest, and the easy identification of noise/artefacts. The isosurfaces were then ray-traced using the open source application Blender [26] . Phylogenetic analyses methods The phylogenetic analyses build on the morphological matrix developed as described in ref. 13 . The morphological data set (201 characters from which 128 are parsimony-informative) was analysed using TNT [11] using equal weights as well as implied weighting [12] under different concavity values ( k =1, 3, 10, 100). Support values were calculated using symmetric resampling [27] , a measure similar to bootstrapping or jackknifing that is less affected by the distortion of frequencies when the characters have different prior weights. The morphological data set was combined with the molecular data set of ref. 13 , and analysed under direct optimization [28] , [29] with POY v. 4 (ref. 30 ) under three parameter sets, including equal weights and two sets with differential indel opening and extension costs (indel opening=3, indel extension=1), one with equal weights for all nucleotide transformations (3,221) and another with differential weights for transversions and transitions (3,211). A search strategy consisting of a timed search (2 h with TBR branch swapping and tree fusing) was used to save an initial set of trees, which were later used as input trees for an analysis with auto_sequence_partition [1] . Nodal support was assessed via parsimony jackknifing [31] , also using auto_sequence_partition and a probability of deletion of 0.36. The number of molecular characters used was 49 fragments (the 4 input 28S ribosomal RNA fragments yielded 8 fragments after auto_sequence_partition; the 10 input 18S rRNA fragments yielded 41 fragments). Additionally, two static alignments were generated, an implied alignment [32] , [33] obtained after the optimal tree from POY (2,065 characters; 466 parsimony-informative), and a multiple sequence alignment obtained in MAFFT (indel cost=3) [34] , [35] (2,001 characters, 471 parsimony-informative). These alignments were analysed in MrBayes v. 3.1.2 (refs 36 , 37 ), both alone and in combination with the morphological data matrix discussed above (10 6 generations retaining 1 tree every 1,000 generations, 4 chains, 15% trees discarded before burn in). For these data sets, we estimated the best-fit model of sequence evolution using jModeltest [38] . In both cases GTR+G+I was selected as the best-fit model. The 18S rRNA and 28S rRNA molecules were each treated as separate partitions in the MrBayes analyses. We analysed the combined data set of the two molecules + morphology for both alignments, assigning different models to morphology and molecules. Justification of character codings The number of characters refers to the morphological matrices published by refs 5 , 13 (the current matrix is included as Supplementary Software 1 ). The eye characters have been recoded for the two stylocellids, according to the newest interpretation of eye homology in Cyphophthalmi [39] , which consider them median eyes, and not lateral eyes as assumed in earlier studies [13] . Due to their size, eyes cannot be unambiguously assigned to the two fossils, and therefore these characters remained as missing data (ch. 1–6). The ocularium (ch. 7) is clearly observed in both fossils, and, in A. scolos , it seems to be of the type of an anterior spine-like projection, as found, for example, in Acuclavella [22] . The shape of the ocularium (ch. 8) has been recoded to reflect possible homology among the forwardly projecting ocular tubercles (whether bifurcating or not) of A. scolos and those of several other Dyspnoi, including the fossil Halitherses grimaldi [5] . Whether the ocularium is smooth or has the typical Eupnoi double row of denticles (ch. 9–10) cannot be observed in either fossil. Cuticular structures (surface ornamentation or pigmentation) as well as other surface structures (setation, tracheal spiracles and their position, or even presence of repugnatorial gland openings) are not observable due to preservation, and therefore are coded as missing data, as are internal anatomy characters, especially those referring to musculature (ch. 220–253) or sperm ultrasturcture (ch. 193–208). The latter two sets of characters from refs 5 , 13 have been inactivated in the current analyses. The total number of characters used is 201, of which 73 are not informative from a cladistic point of view. The palpal tarsal claw (ch. 69), an important character for internal Opiliones phylogeny, has been interpreted as present in M. cronus , and reduced or absent in A. scolos . Other palpal characters are difficult to interpret in A. scolos . In Phalangida leg II is the longest (ch. 70). In the case of our fossil species, in A. scolos , the legs are not completely preserved, but femur II is the longest and we use the length of femora as a proxy for leg length. Data for M. cronus are unclear, and therefore we have left it as missing data. Character 79 has been modified to reflect the diversity in Cyphophthalmi, where some groups have the coxa II fused to coxae III–IV whereas others have it free. In the old data matrix, these two states were combined into one. Sandokanidae (formerly Oncopodidae; Gnomulus and Sandokan ( Oncopus in the old matrix)) have been recoded, as they do not have all coxae free, and instead they have the same state as all other Laniatores. Outgroups have also been recoded accordingly. The presence of an operculum closing the gonostome (ch. 160) is established based on the piece of cuticle inferred between coxae IV, but whether the genital operculum is jointed or not (ch. 161) could not be established. Several characters have been corrected or refined for different terminals. Parasiro has been corrected for spermatopositor sense organ (ch. 174), which is missing in this genus of Cyphophthalmi [40] , and internal genitalic characters for many Laniatores have been coded as missing data (see discussion in ref. 21 ). We have also restricted this analysis to Opiliones and a few potential outgroups, including Xiphosura, Scorpiones, Pseudoscorpiones and Solifugae, and therefore many of the characters used by refs 5 , 13 have become uninformative at this level, but we preferred to keep the original matrix for the sake of simplicity for cross-referencing. How to cite this article: Garwood, R J. et al . Anatomically modern Carboniferous harvestmen demonstrate early cladogenesis and stasis in Opiliones. Nat. Commun. 2:444 doi: 10.1038/ncomms1458 (2011).